Extracellular matrix inhibits structural and functional plasticity of dendritic spines in the adult visual cortex Brain cells are immersed in a complex structure forming the extracellular matrix. The composition of the matrix gradually matures during postnatal development, as the brain circuitry reaches its adult form. The fully developed extracellular environment stabilizes neuronal connectivity and decreases cortical plasticity as highlighted by the demonstration that treatments degrading the matrix are able to restore synaptic plasticity in the adult brain. The mechanisms through which the matrix inhibits cortical plasticity are not fully clarified. Here we show that a prominent component of the matrix, chondroitin sulfate proteoglycans (CSPGs), restrains morphological changes of dendritic spines in the visual cortex of adult mice. By means of in vivo and in vitro two-photon imaging and electrophysiology, we find that after enzymatic digestion of CSPGs, cortical spines become more motile and express a larger degree of structural and functional plasticity. The extracellular matrix (EM) is a crucial determinant of cortical plasticity and the effects of extracellular proteases on the activity-dependent rearrangement of cortical circuitry have long been recognized [1] , [2] , [3] , [4] . The direct link with plasticity is stressed by the activity-regulated maturation of EM [5] , [6] , [7] ending in parallel with the closure of the juvenile critical period of heightened plasticity [6] , [8] . The relationship between critical period closure and EM is reciprocal, as alterations of the EM structure prolong the critical period [9] , [10] and plasticity processes can be partially restored in the adult brain by degradation of the EM [11] , [12] , [13] , [14] , [15] . Key components of the extracellular environment are the chondroitin sulfate proteoglycans (CSPGs): these molecules are formed by a proteic scaffold supporting chondroitin sulfate glycosaminoglycan chains. Initially, it was recognized that CSPGs inhibit axonal sprouting as they are one of the main obstacles to axon regeneration [16] , [17] , [18] . It is now clear that the action of CSPG is multifaceted, as an inhibitory effect of CSPGs on axonal conduction and synaptic transmission in adult rat spinal cord has been recently reported [19] . During development, CSPGs form dense perineuronal nets surrounding parvalbumin-positive fast-spiking interneurons and a less dense, but ubiquitary, diffuse matrix [5] . CSPGs can be degraded by the action of the bacterial enzyme chondroitinase ABC (ChABC) that cleaves the side chains of CSPGs from the proteic core. The injection of ChABC in the visual cortex and in the amygdala has been shown to reactivate juvenile forms of experience-dependent plasticity in adult rodents [12] , [13] . Similarly, the injection of ChABC in the damaged rat spinal cord was also found to improve synaptic plasticity after spinal cord injury [20] . In spite of the accumulating evidence for the role of CSPGs as stabilizers of synaptic connectivity, little is known about the mechanisms underlying the plasticity reinstatement that follows CSPGs degradation. The search for this can be inspired by the inhibitory effects of CSPGs on axonal sprouting that suggest a direct restraining action on the structural remodeling of neurons. Dendritic spines are dynamic structures classically considered as excitatory postsynaptic sites. Intriguingly, dendritic spines are also emerging as inhibitory synaptic sites showing particularly high levels of plasticity [21] , [22] . Morphological plasticity of dendritic spines tightly correlates with the level of cortical plasticity [23] , [24] . Indeed, during circuitry maturation, dendritic spines exhibit spontaneous motility and the formation of filopodial protusions heralds the emergence of novel excitatory synapses [25] . Later on, as the circuitry reaches its adult form, filopodia become very rare, spine motility subsides and connectivity stabilizes. Here we address the hypothesis that CSPGs inhibit dendritic spine motility and functional plasticity thus stabilizing the mature cortex. In vivo imaging in the adult visual cortex showed that the degradation of CSPGs allows for the expression of structural plasticity of dendritic spines and for the appearance of filopodia. Furthermore, removal of CSPGs followed by high frequency activity allows the potentiation of visual responses together with the enlargement of spine heads. These data show that the degradation of CSPGs in the adult visual cortex allows the potentiation of existing synapses at a very short time scale and the formation of new synaptic contacts at a longer time scale. CSPGs restrain motility of dendritic spines in vivo First we tested whether ChABC treatment in the visual cortex of adult mice (older than 70 days) reactivates the basal structural plasticity typical of immature dendritic spines. The occipital cortex of mice expressing green fluorescent protein (GFP) in a sparse set of layer 5 (L5) pyramidal neurons [26] (Thy1-GFP mice) was injected with either ChABC or penicillinase; we show that 3 days later CSPGs were strongly degraded in the ChABC-injected cortex, whereas the control treatment had no effects and the integrity of the perineuronal nets and of the diffuse staining for CSPGs was preserved ( Fig. 1a ). Spine density (0.33±0.12 spines per μm control, 0.34±0.09 spines per μm ChABC; s.d. of the mean) and spine head volume were unaffected by the treatment. 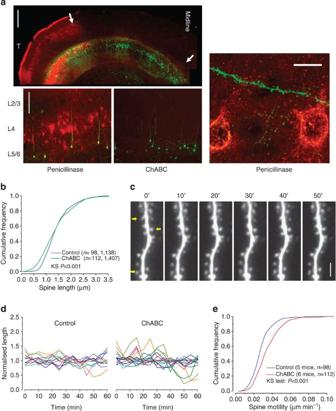Figure 1: CSPG digestion increases spine motility. (a) Cortical coronal section showing GFP fluorescence and WFA fluorescence staining the CSPGs (red). The effect of ChABC treatment is clearly visible in the area between the arrows, where WFA fluorescence is strongly reduced. T indicates the temporal cortex, and the dorsal cortex is at the top of the image. Scale bar, 0.5 mm. The two lower panels show the staining for CSPGs after the injection with penicillinase (left) and ChABC (right). The digestion with ChABC strongly reduces the staining of perineuronal nets and of the CSPG staining diffused in the entire cortex. Scale bar, 200 μm. The right panel shows a detail of perineuronal nets and of the diffused staining after treatment with penicillinase. Scale bar, 15 μm. (b) Cumulative distribution of spine length measured at all temporal points in ChABC-treated and control animals. In parenthesis are indicated the number of spines and the total number of observed temporal points. (c)In vivotime-lapse imaging in a cortex treated with ChABC. Arrows indicates mobile spines. Scale bar, 4 μm. (d) Sample traces showing spine length as a function of time from control and ChABC-treated cortices. (e) Cumulative distribution of spine motility is significantly different between the two groups. Figure 1: CSPG digestion increases spine motility. ( a ) Cortical coronal section showing GFP fluorescence and WFA fluorescence staining the CSPGs (red). The effect of ChABC treatment is clearly visible in the area between the arrows, where WFA fluorescence is strongly reduced. T indicates the temporal cortex, and the dorsal cortex is at the top of the image. Scale bar, 0.5 mm. The two lower panels show the staining for CSPGs after the injection with penicillinase (left) and ChABC (right). The digestion with ChABC strongly reduces the staining of perineuronal nets and of the CSPG staining diffused in the entire cortex. Scale bar, 200 μm. The right panel shows a detail of perineuronal nets and of the diffused staining after treatment with penicillinase. Scale bar, 15 μm. ( b ) Cumulative distribution of spine length measured at all temporal points in ChABC-treated and control animals. In parenthesis are indicated the number of spines and the total number of observed temporal points. ( c ) In vivo time-lapse imaging in a cortex treated with ChABC. Arrows indicates mobile spines. Scale bar, 4 μm. ( d ) Sample traces showing spine length as a function of time from control and ChABC-treated cortices. ( e ) Cumulative distribution of spine motility is significantly different between the two groups. Full size image Spine motility was assessed by imaging a segment of the apical tuft of L5 pyramidal neurons every 5 min for at least 1 h and measuring the spine length at each time point [27] . Motility was measured by computing the rate of change of spine length during each 5 min period. Although the mean spine length was unchanged (1.44±0.54 μm control, 1.40±0.66 μm ChABC; s.d. of the mean), its distribution was wider in ChABC-treated animals ( Fig. 1b ), suggesting a larger variability of this parameter when measured repeatedly during time-lapse sequences ( Fig. 1c ). Indeed, spine motility was enhanced in the cortex treated for 3 days with ChABC ( Fig. 1d ) in comparison to control animals injected with penicillinase. These data show that CSPG degradation caused a marked instability of dendritic spines without changing their number, mean length or volume. Changes in spine motility might be caused by an indirect mechanism involving circuitry modifications and a slowly developing homeostatic regulation of activity. Alternatively, the CSPGs might exert a direct inhibitory effect on the machinery that allows for dendritic spines motility. If the latter hypothesis was true, changes in motility would be apparent rapidly after CSPG digestion. To address this issue, we applied ChABC on the cortical surface for a brief period immediately before imaging. After 1 h of treatment, the degradation of CSPGs was already apparent in correspondence of the craniotomy ( Fig. 2a ). Spine motility was measured in mice after 1 or 3 h of superfusion with either penicillinase or ChABC. 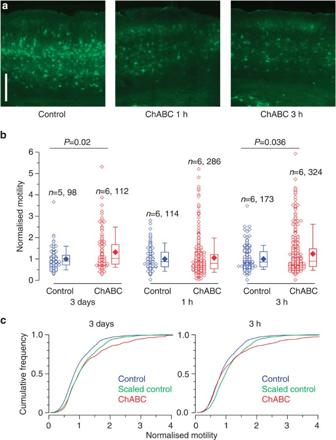Figure 2:In vivoacute treatment with ChABC increases spine motility. (a) WFA staining of the intact EM after superficial treatment with penicillinase (left panel, scale bar 250 μm) and after 1 h (middle panel) and 3 h of ChABC treatment (right panel). (b) The motility of each spine has been normalized to the mean value of the control group of each data point (empty symbols). The mean of each data group is indicated by the solid diamonds, the median by the horizontal bar in the box plot, the box upper and lower edges are the 75% limits and the whiskers the 90% limits. After 1 h of treatment a small group of spines endowed with higher motility is visible. After 3 h the difference is statistically meaningful (Kolmogorov–Smirnov (KS) test,P=0.036, six mice each group, 17 dendrites ChABC, 14 dendrites control). Over each data set is indicated the number of mice employed and the number of imaged spines. (c) Comparison of the cumulative distribution of all spines in control mice (blue line) with the distribution obtained after 3 days or 3 h of ChABC treatment (red, left and right panels, respectively). The green curve is the control distribution, linearly scaled to fit the 3-day treatment midpoint. Figure 2b shows the motility of each imaged spine normalized to the mean of the control of each group: after 1 h of treatment in vivo a population of spines with enhanced motility emerged. After two more hours motility further increased and became very similar to what attained after 3 days of treatment. These data suggest that spines are actively stabilized by local interactions with the perisynaptic components of the EM. As dendritic spines are not specifically associated with perineuronal nets (see Fig. 1a ), it is likely that diffuse CSPGs are responsible for the inhibition of spine motility. From Figures 1d and 2b another interesting data emerges: it seems that the degradation of CSPGs increases motility in a set of spines, whereas others remain relatively more stable. If the treatment with ChABC would equally scale the motility of each spine, one could predict the new motility distribution from the control, by simply scaling the motility of each spine. In the left panel of Fig. 2c we plotted the cumulative distribution of all imaged spines (blue). Then the motility has been scaled (green trace) in order to fit the midpoint of the motility distribution observed after 3 days of treatment (scaling factor 1.16, red trace). Interestingly, the foot of the red distribution is well reproduced by the scaled distribution, indicating that the motility of the more stable spines simply scales linearly after ChABC treatment. However, it is apparent that there is a subgroup of spines representing about 20% of the total, the motility of which scales super-linearly with respect to the control population. A similar effect can be seen after 3 h of treatment (right panel). Figure 2: In vivo acute treatment with ChABC increases spine motility. ( a ) WFA staining of the intact EM after superficial treatment with penicillinase (left panel, scale bar 250 μm) and after 1 h (middle panel) and 3 h of ChABC treatment (right panel). ( b ) The motility of each spine has been normalized to the mean value of the control group of each data point (empty symbols). The mean of each data group is indicated by the solid diamonds, the median by the horizontal bar in the box plot, the box upper and lower edges are the 75% limits and the whiskers the 90% limits. After 1 h of treatment a small group of spines endowed with higher motility is visible. After 3 h the difference is statistically meaningful (Kolmogorov–Smirnov (KS) test, P =0.036, six mice each group, 17 dendrites ChABC, 14 dendrites control). Over each data set is indicated the number of mice employed and the number of imaged spines. ( c ) Comparison of the cumulative distribution of all spines in control mice (blue line) with the distribution obtained after 3 days or 3 h of ChABC treatment (red, left and right panels, respectively). The green curve is the control distribution, linearly scaled to fit the 3-day treatment midpoint. Full size image In vivo long-term potentiation (LTP) after CSPG digestion LTP has been studied in the visual cortex in acute cortical slices where it has been found that LTP of layer 2/3 neurons is developmentally regulated and decreases drastically in the adult cortex at the end of the critical period [28] . Here, we asked whether the enhanced spine motility in ChABC-treated adult mice was accompanied by enhanced functional plasticity of L5 neurons. First, we checked whether high-frequency stimulation (θ-burst) would induce LTP in vivo in layer 5. The apical tuft of L5 pyramidal cells receives a great number of synapses from horizontal connections running in L1 and 2. The activation of a relatively small number of synapses on different branches of the apical tuft is capable of activating an N -methyl- D -aspartate (NMDA) current in the dendrite that successfully propagates to the cell body [29] . Horizontal intracortical connections were stimulated with a 250 μm concentric electrode placed on the cortex surface. The recording electrode was placed in layer 5 at about 0.6 mm under the cortex surface and its tip was centred on the stimulating electrode (see Fig. 3a ). A brief stimulation caused a fast response recorded by the extracellular electrode ( Fig. 3b ): this response is of synaptic origin, as it is blocked by the microinjection of the ionotropic glutammate antagonist kynurate (inset Fig. 3a ). The short latency of the response (ranging from 4 to 8 ms) from the extracellular stimulus correlates with the timing of the NMDA postsynaptic spike evoked in L5 pyramidal neurons [29] and is consistent with a monosynaptic response. After obtaining a stable baseline, we delivered a θ-burst followed by at least 60 min of further recording. The comparison of the responses before and after the θ-burst showed that the amplitude of the putative monosynaptic response was little affected in controls but robustly enhanced in mice treated with ChABC ( Fig. 3b ). 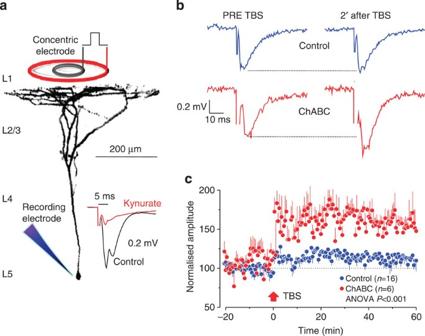Figure 3: Permissive effect of CSPG digestion on visual cortex LTPin vivo. (a) Arrangement of stimulating and recording electrodes. Inset: response to the same stimulus before (black) and after kynurate microinjection 150 μm under the cortical surface (red). (b) Sample of the evoked responses in control (blue) and in ChABC-treated mice (red) before and 2 min after θ-burst. (c) Mean response amplitudes in ChABC-treated (red) and control mice (blue). Theta-burst was delivered at time 0. Bars indicate the error of the mean of each data point. Potentiation is negligible in control mice (one-way analysis of variance (ANOVA),P=0.195) but significant in mice treated with ChABC (one-way ANOVA,P=0.0003, Dunnett’s multiple comparison post tests baseline versus all time points,P<0.01). TBS, θ-burst stimuli. Figure 3: Permissive effect of CSPG digestion on visual cortex LTP in vivo . ( a ) Arrangement of stimulating and recording electrodes. Inset: response to the same stimulus before (black) and after kynurate microinjection 150 μm under the cortical surface (red). ( b ) Sample of the evoked responses in control (blue) and in ChABC-treated mice (red) before and 2 min after θ-burst. ( c ) Mean response amplitudes in ChABC-treated (red) and control mice (blue). Theta-burst was delivered at time 0. Bars indicate the error of the mean of each data point. Potentiation is negligible in control mice (one-way analysis of variance (ANOVA), P =0.195) but significant in mice treated with ChABC (one-way ANOVA, P =0.0003, Dunnett’s multiple comparison post tests baseline versus all time points, P <0.01). TBS, θ-burst stimuli. Full size image Given the geometry of the stimulating electrode, only a minority of synapses is potentiated in these experiments. To study a structural correlate of synaptic potentiation, we need a situation in which a large number of connections is potentiated. Therefore, we tried to induce a less specific and diffused functional potentiation by employing a technique originally described in hippocampal slices. There, it has been demonstrated that a brief incubation of the slice with a solution including picrotoxin (to increase spontaneous activity), rolipram and forskolin (to rise cyclic AMP level), low Mg + and high Ca 2+ (to favour NMDA receptors activation) causes a widespread LTP of CA1 synapses [30] , [31] , [32] . As this protocol has never been attempted on the cortex in vivo , we first characterized the electrical activity induced by the Chem-LTP solution. The upper trace of Fig. 4a shows the extracellular field recording acquired about 20 min after exposure of the cortex surface to Chem-LTP solution. Simultaneous two-photon Ca 2+ imaging in vivo (colored traces) shows that each sharp deflection of the field recording corresponded with a brief synchronous activation of all cortical neurons present in the field. These data indicate that exposure of the cortical surface in vivo to the Chem-LTP solution causes large but brief and stereotyped episodes of intense neuronal firing, similarly to what has been described in hippocampal slices [33] . Amplitude, duration and statistics of this activity were variable among all mice studied but no systematic differences were found between the group treated with ChABC and controls ( Fig. 4b ). Superfusion with the selective NMDA receptor blocker DL-2-amino-5-phosphonopentanoic acid (APV) showed that the late phase of the action potential bursts depended on the activation of NMDA receptors ( Fig. 4c ): this fact is very important because most forms of synaptic plasticity require the activation of these currents. We recorded continuously during treatment to characterize burst frequency: notwithstanding the brief duration of the treatment (10 min) bursting was long lived, which is likely due to the slow diffusion and clearance of the drugs from the intact brain. 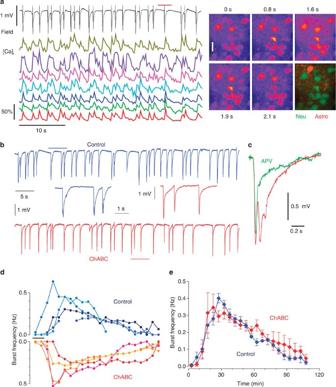Figure 4: Chem-LTPin vivocauses synchronous bursting activity in the visual cortex. (a) The upper trace (black) shows the field recording resulting from perfusion with the Chem-LTP solution. Each large response recorded by the field electrode is associated to the synchronous firing of all neurons in the field, as shown by simultaneous two-photon imaging of calcium concentration. The coloured traces show Ca2+activity of the brightest cells in the field. Images on the right show the Ca2+changes occurring during the burst indicated by the red bar over the field recording. The last image shows the field where neurons are stained by Oregon Green Bapta1, whereas one astrocyte and several processes are stained in red by the dye Sulforhodamine 101. Scale bar, 15 μm. (b) Electrophysiological recordings at the peak of the bursting activity in a control mouse (upper trace) and in a mouse treated with ChABC (lower trace). Insets show typical bursts on an enlarged time scale. (c) Activation of α-amino-3-hydroxy-5-methyl-4-isoxazole propionic acid (AMPA) and NMDA receptors during the synchronous bursts. The red trace show that activation of NMDA receptors supports the late phase of the burst, whereas the early phase, not blocked by APV, is supported by AMPA activation. The red and green traces were recorded immediately before and after superfusion with the NMDA blocker APV. (d) Plots showing the time course of burst frequency. The treatment with the Chem-LTP solution lasts 10 min (black horizontal bar) and bursting activity appears towards the end of treatment. The coloured plots show data from four control mice and four mice treated with ChABC. (e) Average time course of the burst frequency for control and treated mice (mean and s.e.m.). As a measure of the efficacy of the Chem-LTP treatment, we measured the burst frequency: Figure 4d shows that, despite a certain inter-animal variability, the averaged time courses of burst frequency in ChABC-treated and control mice were remarkably similar ( Fig. 4e ). Figure 4: Chem-LTP in vivo causes synchronous bursting activity in the visual cortex. ( a ) The upper trace (black) shows the field recording resulting from perfusion with the Chem-LTP solution. Each large response recorded by the field electrode is associated to the synchronous firing of all neurons in the field, as shown by simultaneous two-photon imaging of calcium concentration. The coloured traces show Ca 2+ activity of the brightest cells in the field. Images on the right show the Ca 2+ changes occurring during the burst indicated by the red bar over the field recording. The last image shows the field where neurons are stained by Oregon Green Bapta1, whereas one astrocyte and several processes are stained in red by the dye Sulforhodamine 101. Scale bar, 15 μm. ( b ) Electrophysiological recordings at the peak of the bursting activity in a control mouse (upper trace) and in a mouse treated with ChABC (lower trace). Insets show typical bursts on an enlarged time scale. ( c ) Activation of α-amino-3-hydroxy-5-methyl-4-isoxazole propionic acid (AMPA) and NMDA receptors during the synchronous bursts. The red trace show that activation of NMDA receptors supports the late phase of the burst, whereas the early phase, not blocked by APV, is supported by AMPA activation. The red and green traces were recorded immediately before and after superfusion with the NMDA blocker APV. ( d ) Plots showing the time course of burst frequency. The treatment with the Chem-LTP solution lasts 10 min (black horizontal bar) and bursting activity appears towards the end of treatment. The coloured plots show data from four control mice and four mice treated with ChABC. ( e ) Average time course of the burst frequency for control and treated mice (mean and s.e.m.). Full size image Next we proceeded to verify whether Chem-LTP was effective in potentiating the physiological activity of the visual cortex. Functional connectivity was estimated by stimulating the eye contralateral to the recorded cortex with a full-field light flash. Light intensity was controlled to cause a half maximal response. Consistently with previous work, no systematic sensitivity differences were found after treatment with ChABC [6] . After recording a stable baseline, the cortex was exposed to the Chem-LTP solution for 10 min followed by several cycles of wash. After treatment it was impossible to estimate the amplitude of the visual-evoked potential (VEP) until all spontaneous bursting subsided. 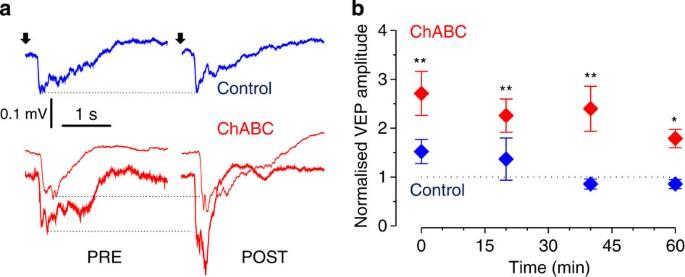Figure 5: Chem-LTP combined with CSPG digestion potentiates visual responses. (a) The evoked potentials to a 100 ms flash (arrowheads) were recorded before cortex superfusion with the Chem-LTP solution (PRE) and 60 min after the end of spontaneous bursting (POST). Data from one control and two mice treated with ChABC are shown. (b) The amplitude of the VEP has been normalized to the amplitude measured before Chem-LTP induction. Time 0 corresponds to the end of the spontaneous bursts. In the control mice, the amplitude of the VEP returned to baseline, whereas a robust potentiation was observed in mice treated with ChABC for 3 days. Data represents mean and s.e. computed by pooling data from four control and four treated mice. **One-wayt-test null hypothesis mean>1,P<0.01. *One-wayt-test null hypothesis mean>1,P<0.02. When all time point are compared the VEP amplitude is significantly larger in treated mice compared with controls (P<0.002 pairedt-test). Figure 5a shows VEPs recorded before Chem-LTP (PRE) and 60 min after the end of spontaneous bursting (POST). Whereas amplitude and shape of VEP was unchanged in the penicillinase-treated mice, it was larger in mice treated with ChABC. In Fig. 5b is reported the mean size of the VEP obtained pooling data from four control and four treated mice. Time 0 refers to the time of the occurrence of the last spontaneous burst. The data demonstrate that visual responses were potentiated in mice treated for 3 days with ChABC, whereas control mice showed no long-lasting potentiation of visual responses. Figure 5: Chem-LTP combined with CSPG digestion potentiates visual responses. ( a ) The evoked potentials to a 100 ms flash (arrowheads) were recorded before cortex superfusion with the Chem-LTP solution (PRE) and 60 min after the end of spontaneous bursting (POST). Data from one control and two mice treated with ChABC are shown. ( b ) The amplitude of the VEP has been normalized to the amplitude measured before Chem-LTP induction. Time 0 corresponds to the end of the spontaneous bursts. In the control mice, the amplitude of the VEP returned to baseline, whereas a robust potentiation was observed in mice treated with ChABC for 3 days. Data represents mean and s.e. computed by pooling data from four control and four treated mice. **One-way t -test null hypothesis mean>1, P <0.01. *One-way t -test null hypothesis mean>1, P <0.02. When all time point are compared the VEP amplitude is significantly larger in treated mice compared with controls ( P <0.002 paired t -test). Full size image Chem-LTP induces rapid structural changes in dendritic spines As a hallmark of excitatory synaptic potentiation is the structural modification of the spine leading to an increased volume of the spine head [24] , [34] , [35] , the next goal was to assess whether Chem-LTP would cause the expression of structural changes of dendritic spines early after treatment, before the time in which we observed potentiation of the visual response. Given the long and variable duration of the spontaneous bursting in vivo , and due to the necessity of imaging dendritic spines at the best possible resolution, we resorted to acute cortical slices. First, we confirmed that the effects of CSPG digestion on dendritic spine motility we observed in vivo held also on acute cortical slices. Time-lapse imaging of slices obtained from control (penicillinase) or ChABC-treated adult mice showed that dendritic spine motility was increased by CSPG digestion, either after a 3-day long treatment ( Fig. 6a , red trace) or after a brief 2 h long incubation of the slice in ChABC ( Fig. 6a , green trace). This brief treatment was equally effective at degrading CSPGs ( Fig. 6b ). A further indication of the destabilization produced by CSPG degradation was the presence of filopodia protruding from dendrites and spine heads ( Fig. 6c ). Filopodia are the telltale sign of spinogenesis, they are abundant during the critical period and disappear during circuitry maturation [25] . The density of filopodia in the adult control mice was only 0.016±0.013 μm −1 (s.d. of the mean) and increased about fivefold to 0.085±0.064 μm −1 after ChABC treatment. Given that the mean density of dendritic spines was unaffected by ChABC, these filopodia are likely to be transient and do not stabilize in mature spines, at least in the time span of these experiments. 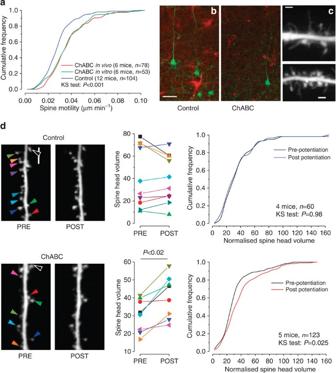Figure 6:In vitrostructural plasticity of dendritic spines. (a) Cumulative distributions of spine motility showing its increase in acute cortical slices both after ChABC treatmentin vivo(red trace) and after 2 h of CSPG digestionin vitro(green trace). (b) CSPG staining (red) of a control slice (left) and after a 2 h digestionin vitro(right). Scale bar, 30 μm. (c) Examples of filopodia and filopodial protusions after 3 days of ChABC treatment. Scale bar, 2 μm. (d) Left panels: sample images taken before and after Chem-LTP (scale bar, 4 μm). Arrowheads point to spines whose volumes are reported with identical colours in the central panels. Here, volumes of spine heads have been measured before and after Chem-LTP. Changes are not significant in control, but are highly significant in the slice from the ChABC-treated mouse (pairedt-test). The volume is measured by an adimensional parameter described inMethods. Right panels show the cumulative distributions of spine head volume before and after Chem-LTP in control (upper graph) and ChABC-treated (lower graph) mice. Figure 6: In vitro structural plasticity of dendritic spines. ( a ) Cumulative distributions of spine motility showing its increase in acute cortical slices both after ChABC treatment in vivo (red trace) and after 2 h of CSPG digestion in vitro (green trace). ( b ) CSPG staining (red) of a control slice (left) and after a 2 h digestion in vitro (right). Scale bar, 30 μm. ( c ) Examples of filopodia and filopodial protusions after 3 days of ChABC treatment. Scale bar, 2 μm. ( d ) Left panels: sample images taken before and after Chem-LTP (scale bar, 4 μm). Arrowheads point to spines whose volumes are reported with identical colours in the central panels. Here, volumes of spine heads have been measured before and after Chem-LTP. Changes are not significant in control, but are highly significant in the slice from the ChABC-treated mouse (paired t -test). The volume is measured by an adimensional parameter described in Methods . Right panels show the cumulative distributions of spine head volume before and after Chem-LTP in control (upper graph) and ChABC-treated (lower graph) mice. Full size image Finally, we induced Chem-LTP in acute cortical slices, obtained from mice treated for 3 days with either ChABC or penicillinase. Imaging performed before and after the induction of Chem-LTP demonstrated a significant increase of spine head volume in slices from ChABC-treated brains, whereas no effects were detected in control slices ( Fig. 6d ), suggesting that the CSPGs degradation allowed for rapid structural changes of dendritic spines. Several mechanisms might contribute to the overall effects caused by digestion of CSPGs on synaptic plasticity, including modulation of ionic conductances, regulation of excitability of fast-spiking interneurons, control of receptor and channel surface localization, just to name a few effectors [14] , [15] . There is no endogenous presence of ChABC in the brain, but there are naturally occurring proteolitic enzymes that include CSPGs in the list of their putative targets. One of these enzymes, MMP-9, was found to drive dendritic spine enlargement and LTP coordinately in hippocampal slices by activating the β-integrin pathway, leading to integrin-dependent cofilin inactivation and actin polymerization [36] . Our data suggest that the increased spine plasticity caused by the degradation of CSPGs leads to an increased susceptibility to activity-dependent potentiation of excitatory connectivity. Intriguingly, in the hippocampus and in the amygdala, the overall sign of the effects of CSPGs degradation goes in the direction of a reduction of LTP and excitatory transmission [13] , [37] . This apparent contradiction might depend on differences in circuitry and on the setting point of the excitation–inhibition balance in the visual cortex. Regardless of this possible regional differences, the increased structural and functional plasticity we described helps in understanding the previous results obtained in the adult visual cortex. If one eye is sutured during the critical period for vision, neuronal responses in the visual cortex are strongly shifted towards the open eye (amblyopia), whereas the closed eye looses the capacity of driving cortical activity [11] . Spine density is affected by this imbalance: in the cortex contralateral to the sutured eye, spine density is decreased compared with the other side dominated by the non-deprived eye. This unbalance of spine density, and of excitatory synaptic input, is maintained through the entire life span even if, in adulthood, the dominant eye is sutured (reverse suture) and therefore there is no recovery of function. However, if the reverse suture is paired with the ChABC treatment, functional amblyopia is partially reverted and spine density is rescued [12] . At the light of our results, we can envision that the recovery of connectivity between the amblyopic eye and the cortex occurs because of the potentiation of existing synapses and because of the formation of new spines. This is also consistent with the observed presence of filopodia after ChABC treatment, in our conditions, the unchanged spine density suggested that, within the brief time window of our experiments (3 days), the filopodia did not stabilize in mature spines. However, the situation might be different in the deprived cortex where the deficit of spines was observed, here it is likely that the digestion of CSPGs allows the formation of spine precursors that successfully mature and stabilize into new spines. Our results suggest that CSPG digestion removes an inhibitory constraint on dendritic spines and allows for the expression of their structural and functional plasticity. Remarkably, it appears that the machinery at the basis of spine motility is constitutively present in spines and it is actively repressed by interactions with the CSPGs. It is conceivable that during ordinary physiological activity, structural plasticity might be opened in the microdomain surrounding a dendritic spine by the activity-dependent release of endogenous proteolitic enzymes, such as MMP9, and that this would account for the residual plasticity still present in adult cortex. These mechanisms might be more important in areas that preserve an higher level of plasticity into adulthood, such as in the hippocampus. The spatially and temporally segregated degradation of EM might emerge as an important modulator of brain circuitry. Animals Two-photon imaging and electrophysiology were performed on homozygous GFP-Thy1 transgenic mice on C57Bl/6 background (mouse line M [26] ). A minority of electrophysiology experiments (electrical LTP) was performed on C57Bl/6 mice: as results were indistinguishable, all the data were pooled together. All mice were 10- to 12-week old. All procedures were approved by and carried out according to the Italian Health Institute and their guidelines. Treatment with chondroitinase Animals were administered with antibiotic (Baytril, 1 ml l −1 , in the drinking water) 1 day before surgical procedure. On the day of surgery, animals were anesthetized with i.p. injection of avertin (0.2 ml per 10 g)/protease-free ChABC (40 U ml −1 , Seikagaku) was diluted in sterile artificial cerebrospinal fluid (ACSF) [6] , [12] . A volume of 1 μl of solution per site at three sites anterior of the visual cortex was delivered at a depth of 500 μm. The skin was sutured and the mouse was allowed to recover. Antibiotic administration continued for 3 days. In control animals, penicillinase (40 U ml −1 , Sigma), a bacterial enzyme lacking endogenous substrate, was administered. In vivo two-photon imaging Imaging was performed 3 days after ChABC (or penicillinase) treatment. Mice were anesthetized with 20% urethane i.p. (ethyl carbamate; Sigma) in saline solution (0.8 ml hg −1 ). The mouse was head-fixed and a craniotomy of 2–3 mm in diameter was drilled over the visual cortex (3–4 mm from the midline). Mice were then mounted under the microscope by means of a support glued to the skull. The support allowed orientation of the cortical surface orthogonally to the optical axis. After imaging, mice were perfused transcardially with 4% paraformaldehyde. Brain sections were cut on a vibratome and incubated with biotin-conjugated lectin Wisteria Floribunda Agglutinin (WFA, Sigma; 1 mg ml −1 ) to label CSPGs. Antigen–antibody binding was revealed with streptavidin fluorescine (Sigma). Acquisition of histological samples was performed at the two-photon microscope and the fluorescence of GFP and fluoresceine was separated by linear spectral decomposition [38] . The ECG signal, picked up by two copper clips placed on the forelimbs, was fed to a differential amplifier (NPI) and then to a threshold discriminator that converted the heart beat waveform into a TTL signal used for imaging synchronization. The two-photon microscope (Ultima IV, Prairie Technology) was equipped with a 10 W laser (Chamaleon Ultra 2, Coherent) tuned at 890 nm that delivered about 30 mW at the sample. Imaging was restricted to the apical dendrites of layer 5 pyramidal neurons in cortical layers 1–2 (50–150 μm below the cortical surface). Imaging was conducted for at least 1 h at an interval of 5 min. Images were acquired with a water immersion lens (Olympus, × 60, numerical aperture: 0.95) at a resolution of 512 × 512 pixels with zoom 4, leading to a field of 50.7 × 50.7 μm and a nominal linear resolution of about 0.1 μm per pixel. The stack step size was 0.75 μm. In vivo two-photon calcium imaging The cortex was bulk loaded with a microinjections of the calcium indicator dye Oregon Green Bapta-1AM (Molecular Probes, Invitrogen) and the selective astrocyte marker Sulforhodamine 101 (Molecular Probes, Invitrogen) [38] . OGB-1AM (50 μg, Molecular Probes, Invitrogen) was dissolved in 4.5 μl DMSO containing Pluronic F-127 and further diluted 1:11 in 45 μl of ACSF to a final concentration of 0.8 mM. The staining solution was sonicated for 10 min at 37 °C, then filtered with 0.20 μm polyvinylidene difluoride/nylon filters and loaded into a borosilicate micropipette (Sutter Instruments, 1–2 μm tip diameter). The micropipette was inserted at an angle into the cortex to the desired depth (150–200 μm) with a micromanipulator (MP285, Sutter Instruments) and the dye was pressure injected (0.5–0.7 bar, 2–3 min) under visual control ( × 10 air objective). Cortical activity was monitored by imaging fluorescence changes at 820 nm. Field potential was recorded in synch with imaging. T-series of fields of variable size were acquired at 3 Hz to detect activity-related somatic calcium signals. Fluorescent cells were imaged at 200–300 mm depth in the cortex. Slice two-photon imaging Brains were sectioned with a vibratome in cold (4 °C) cutting solution containing 132.8 mM NaCl, 3.1 mM KCl, 1 mM CaCl 2 , 2 mM MgCl 2 , 1 mM K 2 HPO 4 , 10 mM HEPES/NaOH, 4 mM NaHCO 3 , 5 mM glucose, 1 mM ascorbic acid, 0.5 mM Myo inositol, 2 mM pyruvic acid and 189.90 mg/ml kynurenic acid. Coronal slices 330 μm thick were prepared from the visual cortex and were allowed to recover in oxygenated cutting solution without kynurenic acid for at least 1 h before the beginning of imaging or pharmacological treatment. In control experiments, we tested synaptic transmission in acute slices between layer 6 and layer 2/3. Upon returning to kynurenic-free solution, synaptic transmission was restored very rapidly (range 3–15 min) both in slices from control mice or from mice treated with ChABC. During imaging, slices were perfused in oxygenated (95% O, 5% CO 2 ) and heated recording medium (132.8 mM NaCl, 3.1 mM KCl, 2 mM CaCl 2 , 1 mM MgCl 2 , 1 mM K 2 HPO 4 , 10 mM HEPES/NaOH, 4 mM NaHCO 3 , 5 mM glucose, 1 mM ascorbic acid, 0.5 mM Myo inositol, 2 mM pyruvic acid). Spine motility experiments were performed 3 days after treatment on a custom-modified FluoView 300 two-photon microscope. In some experiments, in vitro CSPG digestion was carried out by incubating cortical slices from untreated adult mice in oxygenated cutting solution containing 0.1 U ml −1 chondroitinase for 2 h and digestion was assessed at the end of imaging by fixing overnight the slices in 4% paraformaldehyde followed by CSPG staining. Chemical LTP was induced by perfusing the slice for 10 min in Mg-free recording solution modified with the addition of 4 mM CaCl 2 , 0.1 μM rolipram, 50 μM forskolin and 50 μM picrotoxin. This treatment increases the level of cAMP and of electrical activity leading to a tetanic-like stimulation that potentiates a large number of synapses [30] , [31] , [32] , [33] . Imaging was performed on the Prairie microscope. Two-photon image analysis Images were analyzed with ImageJ [27] . The optical sections of each stack were aligned to compensate for mechanical movements with a custom macro in ImageJ. After alignment of the z-stack, the length of each spine was measured on the sections of optimal focus starting from the tip along the neck to the centre of the dendrite. Motility was computed as the average rate of change of the spine length within an interval of 5 min. The spine length was measured in the Z maximum projection from the spine head to the edge of the dendrite. We did not localize the Z position of the spine head: although this underestimates the length of dendritic spines not orthogonal to the optic axis, it does not introduce any specific bias in the relative comparison between treated groups. We found no significant differences for the dendrite diameters and the relative fluctuations during the time-lapse sequences (diameter: control 0.68±0.12 μm; ChABC 0.64±0.11 μm; diameter fluctuation: control 0.013±0.003 μm min −1 ; ChABC 0.015±0.003 μm min −1 ). Spine head volume was computed by normalizing the integrated fluorescence [39] (after background subtraction) from a ROI draw around the spine head with the mean fluorescence of the nearby dendrite. Morphometric measures were performed on the original Z -stacks. For representation purposes, the stacks have been Kalman filtered and projected. The gamma of the image was adjusted to allow a proper visualization of the original 12 bit data on the 8 bit palette. In vivo LTP Adult mice were anesthetized with urethane (0.8 ml hg −1 ) and mounted on a stereotaxic apparatus, oxygenated and body temperature was monitored during the experiment. Extracellular field potentials were recorded in layer 5 of visual cortex with a 1–2 MΩ glass pipette filled with ACSF and inserted at a 45° angle at a 600 μm depth from the surface. Synapses on the apical tufts of pyramidal cells were stimulated by a bipolar platinum/iridium electrode placed on the surface of the cortex vertically above the tip of the recording pipette. The tip of the electrode was stained with DiI (Invitrogen) to confirm the recording position at the end of the experiment. Synaptic transmission was monitored with a run every 30 s. Each run included a stimulation pulse of 0.1 ms. The strength of the stimulation for the following recordings was chosen at 30% of the maximal response. LTP was induced by three θ-burst stimuli at 0.1 Hz. A θ-burst stimuli consisted of ten bursts delivered at 5 Hz, and each burst consisted of five pulses at 100 Hz at a stimulation strength 50 μA lower than that used for test stimulation. The micro-injection of kynurenic acid (10 mM) in layer 2/3 almost totally abolished the synaptic response evoked by the extracellular stimulation confirming the postsynaptic nature of the recorded wave. Field potentials were amplified (NPI Extracellular Amplifier EXT-02F), bandpass filtered (from 0.1 Hz to 1 kHz) and acquired at 2 kHz. Data acquisition and analysis were performed using custom made software. VEP recordings After craniotomy, the dura was removed. A glass micropipette of 1–2 MΩ filled with ACSF was placed at 600 μm depth perpendicular to the cortical surface to record the VEP signal at the level of layer 5. Flash stimuli were produced by a led positioned 10 cm in front of the animal eye contralateral to the recorded cortex. Flash (100 ms) were generated by the VEP acquisition software and were delivered every 10 s. After 10 min, the cortex was washed with ACSF. Field activity was recorded during spontaneous bursting, and the flash was continuously delivered during this period. At the end of spontaneous bursting, VEP amplitude was monitored for at least 1 h. VEP were measured by averaging together at least 20 individual responses. The slow component of spontaneous bursts was NMDA-dependent as it disappeared after the administration of 100 μM NMDA antagonist, APV (Sigma-Aldrich). How to cite this article: de Vivo, L. et al . Extracellular matrix inhibits structural and functional plasticity of dendritic spines in the adult visual cortex. Nat. Commun. 4:1484 doi: 10.1038/ncomms2491 (2013).